Indoleamides are active against drug-resistantMycobacterium tuberculosis Responsible for nearly two million deaths each year, the infectious disease tuberculosis remains a serious global health challenge. The emergence of multidrug- and extensively drug-resistant strains of Mycobacterium tuberculosis confounds control efforts, and new drugs with novel molecular targets are desperately needed. Here we describe lead compounds, the indoleamides, with potent activity against both drug-susceptible and drug-resistant strains of M. tuberculosis by targeting the mycolic acid transporter MmpL3. We identify a single mutation in mmpL3 , which confers high resistance to the indoleamide class while remaining susceptible to currently used first- and second-line tuberculosis drugs, indicating a lack of cross-resistance. Importantly, an indoleamide derivative exhibits dose-dependent antimycobacterial activity when orally administered to M. tuberculosis -infected mice. The bioavailability of the indoleamides, combined with their ability to kill tubercle bacilli, indicates great potential for translational developments of this structure class for the treatment of drug-resistant tuberculosis. Tuberculosis (TB) is a human infectious disease responsible for significant worldwide morbidity and mortality, accountable for an estimated 8.7 million incident cases and 1.4 million deaths in 2011 (ref. 1 ). Although effective therapy exists for TB caused by drug-susceptible Mycobacterium tuberculosis , this therapy requires daily administration of multiple drugs for a minimum of 6 months. Strict adherence to treatment is necessary for successful outcome. However, the intensity and duration of effective therapy challenge patient compliance and thus contribute to treatment failures, leading to increased disease, continued M. tuberculosis transmission and ultimately selection of drug-resistant organisms. The development of drug resistance is especially alarming, as transmission of drug-resistant bacilli can lead to primary infection refractory to standard TB therapy. In 2011, the World Health Organization reported that 3.7% of new TB cases were because of infection with multidrug-resistant (MDR) M. tuberculosis [1] . The tragic development of MDR- and extensively drug-resistant- (XDR-) TB has kindled a worldwide push for the development of new therapy options for this disease, and new drugs are desperately needed to enable effective worldwide TB control. The current World Health Organization-endorsed standard regimen for the treatment of drug-susceptible TB consists of daily rifampin, isoniazid, pyrazinamide and ethambutol for 2 months, followed by 4 months of daily isoniazid and rifampin. This first-line regimen, referred to as the ‘short course’ (as previous treatment regimens ranged from 18 to 24 months in duration), utilizes some of the oldest antibiotics in modern medicine, with isoniazid and pyrazinamide developed in the 1950s and ethambutol and rifampin developed in the 1960s. That the most recent first-line anti-TB drugs are over 50 years old illustrates the paucity of drug development advances in this field. In December 2012, the United States Food and Drug Administration granted accelerated approval of bedaquiline, a diarylquinoline antimycobacterial drug, for the treatment of MDR-TB (infection with M. tuberculosis resistant to rifampin and isoniazid), including XDR-TB (resistance to rifampin, isoniazid, a quinolone and one of the injectable drugs: kanamycin, amikacin or capreomycin), when no other treatment options exist [2] . The Food and Drug Administration approval of bedaquiline is a landmark event in TB chemotherapy, representing the introduction of a new drug class and being the first new TB drug approved in half a century. However, the nature of the approval, being only permitted for use when other treatment options are exhausted, indicates that bedaquiline will be added to otherwise failing drug regimens, and as such it can be anticipated that microbial resistance to this new compound will eventually emerge. Thus, it is imperative that TB drug development efforts continue to push forward. Whole-cell phenotypic high-throughput screening is a powerful tool for evaluation of the antimicrobial activity of compounds in large chemical libraries. Indeed, such high-throughput compound screening with the proxy nonpathogenic organism M. smegmatis identified the diarylquinoline precursor to bedaquiline, which was subsequently optimized for activity against M. tuberculosis [3] . This method has been adapted for direct utility with M. tuberculosis and has led to the identification of a number of promising lead compounds [4] . A recent phenotypic screening of a library of 6,800 compounds identified several chemotypes with anti- M. tuberculosis activity [5] , [6] , [7] , [8] . We synthesized and preliminarily characterized one molecular class, indoleamides, which was active against both drug-susceptible and drug-resistant M. tuberculosis [9] . Here we further characterize three lead compounds from this class both in vitro and in vivo . Our work indicates that these compounds target the mycobacterial membrane protein, large-3 (MmpL3), a mycolic acid transporter, and that the indoleamides are orally bioavailable and effective in vivo in a mouse model of TB, indicating promising translational potential. Indoleamides are active against M. tuberculosis A high-throughput screen of compounds [8] identified a structurally simple indole-2-carboxamide, compound 1 , with activity against M. tuberculosis ( Fig. 1a ). We used the indoleamide scaffold as a basis for the development of structural analogues, which yielded compounds 2 and 3 ( Fig. 1b ). The minimum inhibitory concentration (MIC) values of each of these compounds were determined against different M. tuberculosis strains, including a fully drug-susceptible laboratory reference strain, H37Rv, and five clinical isolates originally obtained from pulmonary TB patients in KwaZulu-Natal, South Africa [7] , [10] . The patient isolates included a drug-susceptible strain (V4207), two confirmed MDR strains (V2475 and KZN494) and two XDR strains (TF274 and R506). As expected, the control strains H37Rv and V4207 were susceptible to the first-line and second-line drugs tested; the MIC values for compounds 1 , 2 and 3 were 0.125–0.25, 0.0156–0.0313 and 0.0039 μg ml −1 , respectively [9] —concentrations that are within a feasible range for translational utility. The MDR strains were resistant to isoniazid and rifampin but susceptible to the second-line drugs tested, and the XDR strains were resistant to all tested drugs [7] . However, the indoleamide compounds exhibited MIC values of ≤1 μg ml −1 for all strains tested, suggesting that this structure class inhibits M. tuberculosis via a novel molecular interaction, and, importantly, that these compounds may be effective against MDR and XDR strains. 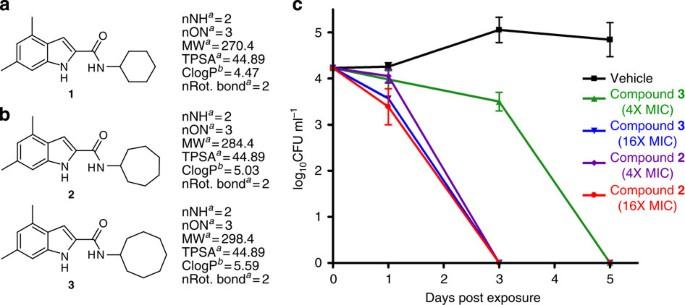Figure 1: Indoleamide compounds are activein vitroagainstMycobacterium tuberculosis. (a) Structure of compound1, the initial hit indoleamide. (b) Structures of compounds2and3, derivatives of compound1. (c)In vitrokill curve ofM. tuberculosisexposed to 4X and 16X MIC of the indoleamide derivative compounds2and3. Data are presented as mean±s.e.m. (n=3). nNH, number of hydrogen bond donors; nON, number of hydrogen bond acceptors; MW, molecular weight; TPSA, topological polar surface area; nRot. bond, number of rotatable bonds; MIC, minimum inhibitory concentration. (a) Calculated using molinspiration online service; (b) Calculated using ChemDraw Ultra 13.0, CambridgeSoft. Figure 1: Indoleamide compounds are active in vitro against Mycobacterium tuberculosis . ( a ) Structure of compound 1 , the initial hit indoleamide. ( b ) Structures of compounds 2 and 3 , derivatives of compound 1 . ( c ) In vitro kill curve of M. tuberculosis exposed to 4X and 16X MIC of the indoleamide derivative compounds 2 and 3 . Data are presented as mean±s.e.m. ( n =3). nNH, number of hydrogen bond donors; nON, number of hydrogen bond acceptors; MW, molecular weight; TPSA, topological polar surface area; nRot. bond, number of rotatable bonds; MIC, minimum inhibitory concentration. ( a ) Calculated using molinspiration online service; ( b ) Calculated using ChemDraw Ultra 13.0, CambridgeSoft. Full size image To further investigate the in vitro antimycobacterial activity of these indoleamide compounds, we determined their minimum bactericidal concentration (MBC) values against the H37Rv strain. For compounds 1 , 2 and 3 , the MBC values were 0.25, 0.0313 and 0.0078 μg ml −1 , respectively. As compounds 2 and 3 exhibited lower MIC values for all M. tuberculosis strains tested than the original hit molecule, we assessed the kill kinetics of these two indoleamide derivatives at concentrations of 4 × and 16 × the MIC with the H37Rv reference strain. The 4 × MIC of both compounds killed at least 4 log 10 colony forming units (CFUs) within 3 or 5 days for compounds 2 and 3 , respectively ( Fig. 1c ), suggesting aggressive bactericidal activity towards M. tuberculosis . Indoleamide physicochemical properties In addition to their promising in vitro bactericidal activity against M. tuberculosis , the indoleamides have physicochemical properties that indicate great potential for absorption and permeation as orally available compounds. Namely, they comply with at least three of the four physicochemical parameters defined by the Lipinski ‘rule-of-five’, which predict aqueous solubility and intestinal permeability [11] . All three indoleamide compounds had less than five hydrogen bond donors, <10 hydrogen bond acceptors and molecular weights <500 g mol −1 ( Fig. 1a,b ). In terms of lipophilicity, compound 1 also had a CLogP value of <5, while compounds 2 and 3 had CLogP values just above 5. The ease of synthesis coupled with the promising physicochemical properties render these compounds attractive for further development as novel anti-TB drugs. Furthermore, we assessed the potential cytotoxicity of our indoleamide compounds on mammalian cells using the Vero cell line. The half maximal inhibitory concentration (IC 50 ) value for Vero cell viability was high for all three tested compounds (>64 μg ml −1 for compounds 1 and 2 , and 16 μg ml −1 for compound 3 ), indicating that they were non-toxic in this model system. Their low MIC values and toxicity profiles resulted in very high selectivity index values, ranging from >256 for compound 1 to >2,048 for compound 2 and 4,000 for compound 3 . mmpL3 mutation confers resistance to indoleamides Initial in vitro experiments and structural analyses indicated that the indoleamides may represent a promising new anti- M. tuberculosis structure class for drug development; however, their bacterial target was unknown. Thus, we selected M. tuberculosis colonies with phenotypic resistance to compound 2 by growing the H37Rv reference strain on 7H10 agar plates containing a range of compound concentrations. We obtained one single CFU on a plate containing compound 2 at 8 × the MIC. This isolate, referred to as IAR2 (indoleamide-resistant, compound 2 ), was able to multiply when inoculated into 7H9 liquid media with the same concentration of compound 2 , indicating that IAR2 was a true resistant mutant selected at a frequency of one in 3 × 10 7 CFUs. To identify mutations associated with resistance, whole-genome sequencing was performed on both the IAR2 and parental H37Rv strains of M. tuberculosis using the Ion Torrent Personal Genome Machine platform. We obtained sequences for >95% of each genome with ~30 × coverage ( Table 1 ), with the average read lengths of 98 and 118 bases for IAR2 and H37Rv, respectively. Relative to the H37Rv parental strain, the IAR2 genome contained a T to A single nucleotide polymorphism (SNP) at position 862 within the Rv0206c gene, encoding for MmpL3, a mycolic acid transporter. This SNP, which was further validated by Sanger sequencing, resulted in a serine to threonine missense mutation at position 288 of the cognate protein ( Fig. 2a ). 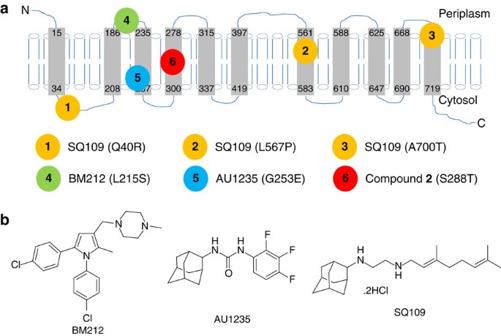Figure 2: MmpL3 is a validated target inMycobacterium tuberculosis. (a) Illustration of the topology of the MmpL3 mycolic acid transporter protein in theM. tuberculosisinner membrane. Coloured circles represent the locations of amino-acid changes associated with resistance to compounds known to target this protein: the diamide SQ109 (ref.15), the pyrrole derivative BM212 (ref.13) and the urea derivative AU1235 (ref.12). (b) Structures of BM212, AU1235 and SQ109. This exact SNP was identified in 14/14 reads at this allele in the IAR2 genome ( Table 2 ). Table 1 Summary statistics of whole genome sequencing. Full size table Figure 2: MmpL3 is a validated target in Mycobacterium tuberculosis . ( a ) Illustration of the topology of the MmpL3 mycolic acid transporter protein in the M. tuberculosis inner membrane. Coloured circles represent the locations of amino-acid changes associated with resistance to compounds known to target this protein: the diamide SQ109 (ref. 15 ), the pyrrole derivative BM212 (ref. 13 ) and the urea derivative AU1235 (ref. 12 ). ( b ) Structures of BM212, AU1235 and SQ109. Full size image Table 2 Single nucleotide polymorphisms identified in the Mycobacterium tuberculosis IAR2 isolate. 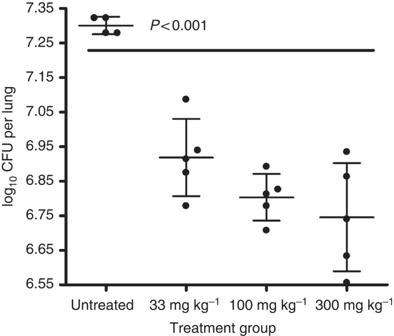Figure 3: The indoleamide compound 3 is active againstM. tuberculosisin a dose-dependent manner duringin vivoinfection of BALB/c mice. Lung CFU counts were assessed 4 weeks after starting daily oral administration of compound3. Each dot represents CFUs from the lungs of an individual mouse, and the bars indicate mean±s.d. CFU counts in each group (n=5 for treated groups andn=4 for untreated control because of one accidental death prematurely). Statistical significance was assessed using the one-way ANOVA with Tukey’s multiple comparison test. CFU, colony forming unit. Full size table We then re-evaluated the MIC values of each of our indoleamide compounds for the IAR2 mutant and found the MIC to be much higher than the parental H37Rv strain ( Table 3 ). The MIC upshift of this structure class ranged from 32- to 64-fold for compounds 2 and 3 to ≥1,024-fold for compound 1 , suggesting that MmpL3, a mycolic acid transporter, is the target of the indoleamide compounds. Interestingly, in the last year, three different compounds have been reported to also target MmpL3: the urea derivative AU1235 (ref. 12 ), the pyrrole derivative BM212 (refs 13 , 14 ) and the diamine SQ109 (ref. 15 ) ( Fig. 2b ). We therefore determined the MIC values of these three compounds for the IAR2 mutant and found that the MIC for each compound was higher for IAR2 than for the parental H37Rv strain ( Table 3 ). Table 3 MIC of indoleamides and three additional compounds reported to target the MmpL3 mycolic acid transporter. Full size table The IAR2 mutant is not cross-resistant to TB drugs To assess the novelty of the microbial target of the indoleamide scaffold and the possible translational utility of this class of compounds for the treatment of both drug-susceptible and drug-resistant TB, we determined the MIC values of commonly used first-line (isoniazid, rifampin and ethambutol) and second-line (levofloxacin, moxifloxacin, kanamycin, capreomycin and amikacin) TB drugs on the IAR2 mutant and its H37Rv parental strain. All of the tested drugs exhibited the same MIC values for IAR2 as for H37Rv (except for rifampin, which actually had a lower MIC value for the mutant strain, Table 3 ). These results demonstrate that MmpL3 may be a validated molecular target in M. tuberculosis and that the S288T mutation in this target does not result in any cross-resistance to drugs currently used for TB treatment. An indoleamide inhibits M. tuberculosis growth in vivo All of the in vitro experiments indicated that our indoleamide compounds may represent a new structure class active against a membrane transporter in M. tuberculosis (MmpL3) that is not targeted by existing TB drugs, prompting evaluation of the activity during in vivo infection. As compound 3 exhibited a dose-dependent mycobactericidal effect in vitro , we analysed the effect of administration of this most potent compound to M. tuberculosis -infected mice. Female BALB/c mice were infected by aerosol with M. tuberculosis H37Rv (day 1 implantation of 3.0 log 10 CFU per lung), and 2 weeks after infection, when the bacterial burden was 6.5 log 10 CFU per lung, compound 3 was administered daily to the mice by oral gavage at doses of 33, 100 and 300 mg kg −1 . After 4 weeks of treatment, the lung CFU counts were significantly lower in mice receiving any dose of compound 3 compared with untreated mice, and the bacterial burden in the lungs declined in a dose-dependent manner ( Fig. 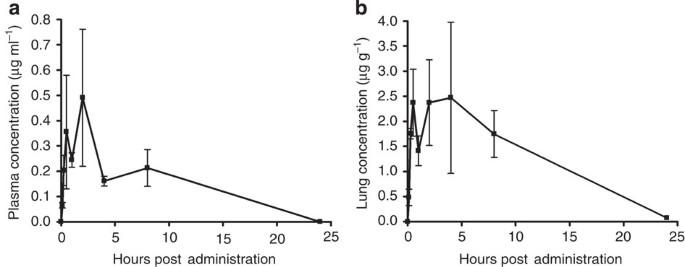Figure 4: Pharmacokinetic analysis of compound 3 in female BALB/c mice. (a) Concentration in plasma and (b) concentration in the lung following a single 100 mg kg−1dose administered by oral gavage. Data are presented as mean±s.e.m. (n=3). 3 ; Table 4 ). Pharmacokinetic studies indicate that the 100 mg kg −1 dose results in a maximum concentration of 0.49 μg ml −1 in plasma and 2.47 μg g −1 in the lungs ( Table 5 ), well above the in vitro MIC value of 0.0039 μg ml −1 . Furthermore, in both the plasma and the lung, the concentration of compound 3 remained above the MIC for nearly 24 h ( Fig. 4 ). These data indicate that compound 3 is orally bioavailable in the mice and is active against M. tuberculosis in vivo . Figure 3: The indoleamide compound 3 is active against M. tuberculosis in a dose-dependent manner during in vivo infection of BALB/c mice. Lung CFU counts were assessed 4 weeks after starting daily oral administration of compound 3 . Each dot represents CFUs from the lungs of an individual mouse, and the bars indicate mean±s.d. CFU counts in each group ( n =5 for treated groups and n =4 for untreated control because of one accidental death prematurely). Statistical significance was assessed using the one-way ANOVA with Tukey’s multiple comparison test. CFU, colony forming unit. Full size image Table 4 Bacterial burden in mouse lungs. Full size table Table 5 In vivo pharmacokinetic parameters of compound 3 in female BALB/c mice. Full size table Figure 4: Pharmacokinetic analysis of compound 3 in female BALB/c mice. ( a ) Concentration in plasma and ( b ) concentration in the lung following a single 100 mg kg −1 dose administered by oral gavage. Data are presented as mean±s.e.m. ( n =3). Full size image New drugs for the treatment of TB, including those that are effective against MDR- and XDR-TB, are greatly needed in the global effort to control this deadly disease. Whole-cell phenotypic screening has been demonstrated to be an effective method for the identification of novel structural classes of antimicrobial compounds and in fact has proven more likely to generate lead compounds than rationale drug-design approaches [11] . However, appreciable limitations of this method include the lack of information regarding the target(s) of compounds, in vivo availability and tolerability. While the former limitation does not necessarily preclude the forward development of hit compounds, knowledge of the target(s) allows for effective lead optimization, providing a molecular basis for structure–activity relationship analyses and also indicating potential pathways for toxic activity within eukaryotic cells. The latter limitation is critical, and the demonstration of safe in vivo activity of a compound is absolutely essential for its continued development. Here we describe a new structural class, the indoleamides, with promising activity against M. tuberculosis . Importantly, we have both identified the mycobacterial target and demonstrated in vivo availability and efficacy of this chemotype, overcoming two of the major hurdles in preclinical drug development. Using the original hit compound 1 ( Fig. 1a ) identified from high-throughput screening, as well as two additional derivatives of this molecule (compounds 2 and 3 , Fig. 1b ), we demonstrated that these indoleamides were highly active against drug-susceptible, MDR and XDR M. tuberculosis strains [9] , suggesting that these molecular entities may interact with a novel mycobacterial target. Indeed, the whole-genome sequencing of an in vitro -selected mutant resistant to compound 2 revealed a mutation in the gene encoding for the mycolic acid transporter MmpL3 ( Fig. 2a ). Although currently not the known target of any licensed drug, MmpL3 has recently been identified as the target of several antimycobacterial compounds, strongly indicating that this transporter represents a bona fide target for anti-TB drug development. Our indoleamide-resistant mutant, IAR2, exhibited full sensitivity to currently used first- and second-line TB drugs ( Table 3 ), indicating a lack of cross-resistance. Importantly, we also demonstrated that an indoleamide derivative (compound 3 ) was orally bioavailable and active against M. tuberculosis in a mouse model of TB ( Fig. 3 ). These studies suggest that the indoleamide structural class represents a valuable source of possible agents effective against both drug-susceptible and drug-resistant TB. Interestingly, the indoleamide structural class was also identified to be active on M. tuberculosis by an independent group [16] , verifying the antitubercular property of this class. The mycobacterial MmpL proteins belong to the resistance, nodulation and (cell) division (RND) family of membrane transporters [17] . RND family proteins are known to mediate the transport of a wide variety of substrates, including antimicrobial compounds, across cell membranes and are also established as virulence factors for several bacterial pathogens [18] . M. tuberculosis strains encode up to 14 known MmpL family proteins, of which MmpL3 has been the least characterized because of difficulties in deleting its cognate gene, suggesting essentiality for the microorganism [17] , [19] , [20] . Interestingly, MmpL3 has recently been identified as the target for a number of structurally distinct compounds: the pyrrole derivative BM212 (refs 13 , 14 ), the urea derivatives AU1235 (ref. 12 ) and 1-adamantyl-3-heteroaryl ureas [21] , the diamine SQ109 (ref. 15 ) ( Fig. 2b ) and tetrahydropyrazolo[1,5- a ]pyrimidine-3-carboxamide and N- benzyl-6′,7′-dihydrospiro[piperidine-4,4′-thieno[3,2- c ]pyran] analogues [22] ; these studies have also revealed a role for MmpL3 in the transport of mycolic acids across the M. tuberculosis cell membrane. The molecular mechanisms involved in mycolic acid synthesis and assembly of the cell wall are well-appreciated molecular targets for both growth inhibition and killing of mycobacteria, being affected by the key TB drugs including isoniazid and ethambutol [23] . Thus, our finding that the indoleamide scaffold targets MmpL3 further corroborates the accumulating evidence that compound-based interactions with this protein interfere with M. tuberculosis growth. That we were able to target MmpL3 with an orally bioavailable compound suggests real translational possibility for the indoleamide structural class. Our indoleamide-resistant M. tuberculosis strain, IAR2, was derived in vitro in the presence of compound 2 , and we found that this strain contained a SNP in the gene encoding for MmpL3, resulting in an S288T amino-acid change, which is predicted to occur in the fourth transmembrane domain of the transporter ( Fig. 2a ). This alteration in MmpL3 was associated with decreased susceptibility to all of the indoleamides (compounds 1 , 2 and 3 ), and interestingly also resulted in decreased susceptibility to the other known MmpL3-targeting compounds SQ109 and AU1235, and possibly BM212, as the increase in MIC value was only twofold ( Table 3 ). In vitro -selected M. tuberculosis mutants resistant to these compounds were found to have different MmpL3-associated mutations, as illustrated in Fig. 2a . Thus, it is intriguing that the S288T mutations conferred resistance to these compounds. However, it is possible that this amino-acid substitution in the transmembrane domain of MmpL3 alters the transporter structure in such a way that SQ109, BM212 and AU1235 cannot adequately access their targets within the protein. It would be of great interest to determine whether the M. tuberculosis strains resistant to these compounds are also resistant to the indoleamides. Certainly, our work provides further validation that MmpL3 is a viable target for anti-TB drug development. Furthermore, we demonstrated that the IAR2 mutant was fully susceptible to the commonly used first- and second-line TB drugs ( Table 3 ). Considering that the AU1235-resistant mutant described by Grzegorzewicz et al. [12] was also susceptible to the currently approved TB drugs, our data strongly suggest that targeting MmpL3 is a valid strategy for the treatment of drug-resistant TB. A key finding in our work is that the indoleamide structure class exhibited oral bioavailability and effectiveness in vivo in a mouse model of TB, thus demonstrating that these two large obstacles of high-throughput screening-based drug development can likely be overcome with members of this structure class. Moreover, lead optimization could result in increased in vivo activity of this group. The compound SQ109, which was identified from a phenotypic compound screen of a directed combinatorial library, has been shown to also be a very promising agent that also targets MmpL3, that was proven to be safe and well-tolerated in Phase I and early Phase II clinical trials [24] , [25] . Our identification of an additional MmpL3-targeting class of compounds considerably bolsters the SQ109 work and could be developed in a complementary context, providing another effective, orally available option for TB treatment. Furthermore, it would be incredibly beneficial to examine whether combination of these two compounds could provide a synergistic effect for the complete inhibition of this essential target. In summary, we have identified a novel structural class, the indoleamides, which interacts with a validated target in M. tuberculosis , the MmpL3 transporter, and show vigorous activity against both drug-susceptible and drug-resistant (including MDR and XDR) M. tuberculosis strains. Our studies build upon and complement new and exciting findings in this field and strongly suggest that the indoleamides have serious translational potential for development into a real tool for TB treatment and control. Chemistry Starting materials, reagents and solvents were purchased from commercial suppliers and used without further purification unless otherwise stated. Anhydrous dichloromethane (CH 2 Cl 2 ) was obtained by distillation over calcium hydride. Thin layer chromatography (TLC) was performed with Merck 60 F254 silica gel plates. Flash chromatography was performed using CombiFlash Rf system with RediSep columns or alternatively using Merck silica gel (40–60 mesh). Final compounds were purified by preparative high-performance liquid chromatography (HPLC) using an ACE 5-AQ (21.2 mm × 150 mm) column, with detection at 254 and 280 nm on a Shimadzu SCL-10A VP detector, flow rate=17.0 ml min −1 . Method 1: 50–100% CH 3 OH/H 2 O in 30 min; 100% CH 3 OH in 5 min; 100–50% CH 3 OH/H 2 O in 4 min. Method 2: 25–100% CH 3 OH/H 2 O in 30 min; 100% CH 3 OH in 5 min; 100–25% CH 3 OH/H 2 O in 4 min. Method 3 : 15–100% CH 3 OH/ H 2 O in 30 min; 100% CH 3 OH in 5 min; 100–15% CH 3 OH/H 2 O in 4 min. Both solvents contained 0.05 vol % of trifluoroacetic acid (TFA). The purities of all final compounds were determined to be >95% using the Agilent 1100 HPLC system with a Synergi 4-μm Hydro-RP 80A column, on a variable wavelength detector G1314A. Sequence: Flow rate=1.4 ml min −1 ; gradient elution over 20 min, from 30% CH 3 OH-H 2 O to 100% CH 3 OH (both solvents contained 0.05 vol % of TFA). 1 H nuclear magnetic resonance (NMR) and 13 C NMR spectra were recorded on a Bruker spectrometer at 400 and 100 MHz, respectively, with tetramethylsilane (TMS) as an internal standard. 1 H and 13 C chemical shifts are reported in δ (parts per million). Standard abbreviations indicating multiplicity were used as follows: s=singlet, d=doublet, dd=doublet of doublets, t=triplet, q=quadruplet, m=multiplet and br=broad. High-resolution mass spectroscopy (HRMS) experiments were performed on Q-TOF-2TM instrument (Micromass). Synthesis of compounds The target compounds were synthesized by employing an efficient amide-coupling protocol. To a solution of 4,6-dimethyl-1 H -indole-2-carboxylic acid (1 equiv) in anhydrous CH 2 Cl 2 (4 ml mmol −1 ) at room temperature were added anhydrous hydroxybenzotriazole (HOBt, 1 equiv) and 1-ethyl-3-(3-dimethylaminopropyl) carbodiimide hydrochloride (EDAC·HCl, 1 equiv) under an argon atmosphere. After stirring for 10 min, the appropriate substituted amine (1 equiv) and triethylamine (1.5 equiv) were added, and the reaction mixture was stirred at room temperature until disappearance of the starting material (usually 12–16 h). After this time, water (2 ml) was added, and the mixture was extracted with ethyl acetate (EtOAc) (3 × 10 ml), the combined organic layers were separated, washed with brine, dried over anhydrous sodium sulfate, filtered and concentrated under reduced pressure. The residue was subjected to flash chromatography (EtOAc–hexane 1:4) to obtain the indole-2-carboxamides in good yields prior to further HPLC purification. Structure–activity relationships of these compounds are reported in Onajole et al. [9] Bacterial strains Wild-type M. tuberculosis H37Rv lab strain was obtained from the Johns Hopkins Center for Tuberculosis Research laboratory stocks. The KwaZulu-Natal clinical isolates used in this study were a kind gift from Dr William R. Jacobs, Jr, at the Albert Einstein College of Medicine. MIC and MBC assays MIC was determined using microplate alamar blue assay [7] , [8] . Plates were then read using a fluorescence microplate reader at 544 ex/590 em. Percentage inhibition was calculated based on the relative fluorescence units and the minimum concentration that resulted in at least 90% inhibition was identified as MIC. For this assay, 7H9 broth without Tween-80 was used as the assay media. For MIC and MBC determination using tube-broth dilution methods, compounds 1 , 2 and 3 were twofold serially diluted at a volume of 2.5 ml in 7H9 without Tween-80. Mid-log phase H37Rv culture was diluted, and 0.1 ml of the diluted culture containing 10 5 CFUs was added to each of the assay tubes. Media control, positive control (isoniazid) and growth control (no compound) were included. Tubes were incubated at 37 °C. On days 7 and 14, pellet formation was observed and recorded and the minimum concentration that prevented pellet formation was identified as MIC. The end point CFUs per tube for the treatment was determined on the tubes that did not show pellet on Day 14. The minimum concentration that killed 99% of the inoculum was identified as the MBC. Kill kinetic assay M. tuberculosis H37Rv culture was diluted to an OD 600 of 0.001 and then divided to five of 10 ml aliquots and supplemented with a final concentration of 0.016 μg ml −1 (4 × MIC) or 0.064 μg ml −1 (16 × MIC) of compound 3 or 0.125 μg ml −1 (4 × MIC) or 0.5 μg ml −1 (16 × MIC) of compound 2 . On days 0, 1, 3 and 5, cultures were diluted and plated. CFUs per ml were enumerated after 4 weeks of incubation. Cytotoxicity assay Vero cell linage (ATCC CCL-81) was grown in Dulbecco’s Modified Eagle Medium (DMEM) containing 10% fetal bovine serum (FBS). Flat-bottomed 96-well plate was seeded with 4 × 10 4 cells. The plate was incubated at 37 °C with 5% CO 2 for 16 h. For compound preparation, twofold serial dilution was made using a deep-well block using DMEM containing 5% FBS with a volume of 200 μl. Culture media was replaced with 160 μl of the compound-containing media, with 100% DMSO as positive (100% kill) control and media only as blank (100% viability) control. The plate was incubated for 72 h and then washed twice with PBS before adding 100 μl of DMEM with 5% FBS medium freshly mixed with 10% alamar blue. The plate was incubated for 2 h and then immediately read with a fluorescence microplate reader at 544Ex/590 Em. The minimum concentration that killed at least 50% of the cells was identified as IC 50 . Selection of indoleamide-resistant mutant To select for resistance, 7H10 agar plates containing 2 × , 4 × , 8 × and 16 × MIC of compound 2 were prepared. Late log phase M. tuberculosis H37Rv culture (OD 600 ~1.0) was spread on these plates and incubated at 37 °C for 4 weeks. Colonies were recovered and propagated in 7H9 broth containing correspondent level of the compound. Deep sequencing and target identification Genomic DNA was isolated from both the parental wild-type (H37Rv) and the resistant mutant (IAR2) strain by using the lysozyme and cetyltrimethylammonium bromide in glucose-tris-EDTA buffer methods. Five microgram DNA was subjected to Covaris S2 DNA shearing system to prepare DNA fragments. The library was prepared and enriched by using the Ion OneTouch and Ion OneTouch Template Kit systems. Enriched template-positive Ion Sphere Particles were sequenced using the Ion Torrent Personal Genome Machine following the Ion 316 Chip protocol and the Ion Sequencing Kit User Guide v2.0 (Life Technologies). After on-machine filtering, all reads were tempted to be aligned to the published M. tuberculosis H37Rv sequence [26] by using the Burrows-Wheeler Aligner algorithms [27] . SNPs were analysed and called by the GATK package. Mouse aerosol infection and monotherapy model Four- to-six-week-old female BALB/c mice were aerosol-infected with M. tuberculosis H37Rv. From 14 days after infection, group of five mice were treated with 33.3, 100 and 300 mg kg −1 of compound 3 by oral gavage, daily (5 days per week). Isoniazid at 10 mg kg −1 was administered as positive control. Infected but untreated mice were negative control. On days −13, 0, 7, 14 and 28 from treatment start, five mice from each treatment were killed and the lungs were removed. The lungs were bead-beaten to homogenate, diluted and plated on 7H11 selective agar plates. All animal procedures were approved by the Institutional Animal Care and Use Committee of the Johns Hopkins University School of Medicine. In vivo pharmacokinetic evaluation Female BALB/c mice (20 g each, Charles River Laboratories) were given a single dose of compound 3 at 100 mg kg −1 by oral gavage in a volume of 0.2 ml. At 0.125, 0.25, 0.5, 1, 2, 4, 8 and 24 h after compound administration, animals ( n =3 per time point) were euthanized and cardiac blood (~0.7 ml) was collected. Mouse lungs were removed, weighed and stored at −80 °C. Plasma was separated using centrifugation at 12,000 × g for 20 min at 4 °C and stored at −80 °C. Mouse lungs were homogenized by bead-beating in 0.5 ml of liquid chromatography/mass spectrometry (LC/MS) water and supernatants were recovered using centrifugation at 4 °C for 20 min. Concentrations of compound 3 in plasma and lung homogenate supernatants were analysed with LC-tandem MS (LC-MS/MS, AB SCIEX QTRAP 5500 system) with compound 2 as internal standard. MS detection of mass transitions 299.01/146.1 and 299.01/131.1 was carried out. Concentration calculation was performed with MultiQuant Software (Version 2.1, AB SCIEX). The pharmacokinetic profile of the test compound was analysed from plasma and lung concentration–time data after oral administration. The peak concentration ( C max ), the time of peak ( T max ), and the area under the concentration curve from time 0 to 24 h (AUC 0–24 ) were calculated by using GraphPad Prism 4. Accession codes: The genomic deep sequencing data have been deposited in the NCBI Trace and Short Read Archives under accession code SRP030413 . How to cite this article: Lun, S. et al. Indoleamides are active against drug-resistant Mycobacterium tuberculosis . Nat. Commun. 4:2907 doi: 10.1038/ncomms3907 (2013).